The polymeric mucin Muc5ac is required for allergic airway hyperreactivity In asthma, airflow obstruction is thought to result primarily from inflammation-triggered airway smooth muscle (ASM) contraction. However, anti-inflammatory and smooth muscle-relaxing treatments are often temporary or ineffective. Overproduction of the mucin MUC5AC is an additional disease feature that, while strongly associated pathologically, is poorly understood functionally. Here we show that Muc5ac is a central effector of allergic inflammation that is required for airway hyperreactivity (AHR) to methacholine (MCh). In mice bred on two well-characterized strain backgrounds (C57BL/6 and BALB/c) and exposed to two separate allergic stimuli (ovalbumin and Aspergillus extract), genetic removal of Muc5ac abolishes AHR. Residual MCh responses are identical to unchallenged controls, and although inflammation remains intact, heterogeneous mucous occlusion decreases by 74%. Thus, whereas inflammatory effects on ASM alone are insufficient for AHR, Muc5ac-mediated plugging is an essential mechanism. Inhibiting MUC5AC may be effective for treating asthma and other lung diseases where it is also overproduced. Asthma is a major health problem. Worldwide, it affects more than 300 million people. In the United States, it affects ~10 million and costs $50–60 billion per year to treat. Asthma is characterized by airflow obstruction and structural changes associated with acute and chronic lung inflammation. Accordingly, the most widely used therapies are bronchodilators and anti-inflammatory agents [1] . However, treatment results are often temporary or incomplete, and alternative strategies are lacking. We propose that this is due to an incomplete understanding of the mechanisms by which airflow obstruction and symptoms of dyspnoea, cough and wheezing are caused by the combined effects of inflammation, bronchoconstriction and additional non-contractile mechanisms. Non-contractile factors include airway wall thickening due to oedema and structural remodelling [2] , loss of airway liquid surface tension due to plasma extravasation and fibrin accumulation [3] and airway occlusion due to mucus hypersecretion [4] . With even just a small amount of airway smooth muscle (ASM) constriction, these non-contractile components can geometrically amplify airway resistance and increase the propensity for airways to close [5] , [6] , [7] , [8] . In human asthma and in animal models, mucin overproduction and hypersecretion are prominent pathological findings [9] , [10] , [11] , [12] , [13] , [14] . In its most severe setting—fatal asthma—autopsy studies show that patients die from severe airflow obstruction caused by bronchoconstriction coupled with widespread mucous plugging [15] , [16] , [17] . Even in mild to moderate asthma, where there is minimal baseline airflow limitation, patients respond to the inhaled cholinergic agonist methacholine (MCh) with exaggerated obstruction. Existing dogma labels this airway hyperreactivity (AHR) to MCh as resulting from excessive ASM contraction [1] . Thus, unlike fatal asthma, where mucus hypersecretion is well recognized, in non-fatal exacerbations the potential obstructive role of mucus has been largely overlooked [1] . In fact, in mild to moderate disease, mucin overproduction is highly prevalent [12] , and the genomic region on chromosome 11p15 that encodes airway polymeric mucins is associated with AHR [18] . Furthermore, mucin overproduction and changes in its biochemical/biophysical properties correlate with asthma exacerbations [4] , [19] , [20] . These associations in humans are supported in animal models where mucin overproduction and AHR to MCh are both induced, and where in addition to causing ASM contraction, MCh is also known to cause mucin secretion [21] , [22] . Thus, the obstructive effects of ASM contraction may be amplified by acute thickening of mucus on airway surfaces. While these associations are strong, establishing the causative significance of mucus secretion in asthma has been hampered by a lack of experimental evidence and the absence of effective clinical interventions that target the chief glycoprotein components of airway mucus, the secreted polymeric mucins MUC5AC and MUC5B. MUC5B predominates in healthy human lungs, and its levels in asthma remain stable or in some cases decrease [10] , [12] , [23] . On the other hand, MUC5AC levels in asthma increase significantly and consistently [4] , [10] , [12] , [13] . Mice display similar tightly controlled expression patterns: High baseline Muc5b gene expression remains stable following antigen challenge while low baseline Muc5ac gene expression increases markedly [24] . Furthermore, whereas Muc5b is required for airway homeostasis and anti-bacterial defence, Muc5ac is not essential for these functions [25] , and in lung injury Muc5ac is actually detrimental [26] . These findings implicate Muc5ac as a deleterious and dispensable glycoprotein component of airway mucus. Thus, it is suitable to investigate as a potential target for reducing obstruction in asthma. In allergic asthma, a biphasic response occurs after allergen inhalation. Acutely, IgE crosslinking induces mast cell and basophil histamine release, causing a brief episode of airflow obstruction (what is most commonly thought of as an ‘asthma attack’). The acute early-phase response lasts a few minutes to a few hours, and it is followed by a late-phase response that lasts for several hours to several days. Clinically, the late phase is considered to be the main driver of disease progression [27] . Accordingly, even after baseline lung function is restored following an acute asthma episode, the ensuing late phase displays sustained pathophysiology hallmarked by AHR to inhaled agonists such as MCh, inflammation characterized by recruitment of eosinophils and interleukin (IL)-13-producing type-2 T helper cells, and airway remodelling linked to induced MUC5AC production [28] . MUC5AC/Muc5ac induction is a well-characterized epithelial response to allergic (type 2) inflammation. IL-13 has been implicated in the pathogenesis of human asthma [29] and in animal models [30] , [31] . However, compared with its reported effects on leukocytes [32] or ASM [33] , the relative importance of IL-13 signalling in epithelia [34] and the mechanisms by which it elicits asthma-like pathophysiology are unclear. MUC5AC/Muc5ac gene expression is induced by IL-13 through direct stimulation of airway epithelial cells [24] , [30] , [31] , [34] , [35] , [36] . In mice, Muc5ac expression is central to the allergic mucous phenotype. It is induced maximally 48–72 h after antigen challenge [24] , times that are concordant with late-phase human asthma. We thus hypothesized that eliminating this type-2 inflammation effector would protect against asthma-like disease in mice. Here we show the functional significance of Muc5ac in allergic AHR, inflammation and mucus obstruction. In Muc5ac −/− mice [37] , we demonstrate that even in the presence of ongoing inflammation, significantly reduced heterogeneous mucous plugging abolishes AHR. Muc5ac is a major polymeric mucin in allergic mouse lungs In wild-type (WT) mice, immunohistochemical analyses demonstrated constitutive Muc5b production that was similar in healthy and ovalbumin (OVA)-sensitized and -challenged airways ( Fig. 1a,b ). OVA challenge induced Muc5ac protein and alcian blue-periodic acid Schiff’s positive glycoconjugate production ( Fig. 1a,b ), which were marked by a ~400-fold increase in Muc5ac transcripts ( Fig. 1c ). In OVA-challenged Muc5ac −/− mice, Muc5ac transcripts were absent ( Fig. 1c ), and bronchial epithelial mucin content was significantly reduced ( Fig. 1d,e ). We thus examined the development of allergic asthma-like phenotypes in Muc5ac −/− mice. 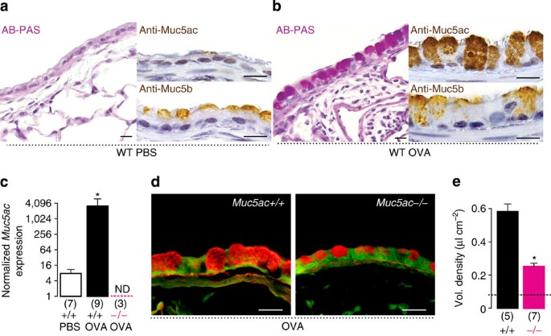Figure 1:Mucous metaplasia is significantly reduced inMuc5ac−/−airways. (aandb) Mucin production in saline- (a) and OVA- (b) challenged WT mice. AB-PAS, anti-Muc5ac and anti-Muc5b staining shows upregulated Muc5ac and sustained Muc5b in allergic airways. (c–e)Muc5acmessenger RNA increased 383-fold in OVA-challenged WT mice (+/+), but it was undetectable inMuc5acknockout (−/−) mice (c), resulting in a 67% reduction in mucous metaplasia detected by periodic acid fluorescent Schiff’s staining (dande). Scale bars, 20 μm (a,b,d). Mean, s.e.m. (cande). *P<0.05 (one-tailed) by a unpairedt-test (cande), with Welch’s correction for unequal variances inc. ND, not detected. Numbers in parentheses, ‘N’ mice. ‘Vol.’, volume. Dashed line ine, baseline in saline-challenged WT mice. Figure 1: Mucous metaplasia is significantly reduced in Muc5ac − / − airways. ( a and b ) Mucin production in saline- ( a ) and OVA- ( b ) challenged WT mice. AB-PAS, anti-Muc5ac and anti-Muc5b staining shows upregulated Muc5ac and sustained Muc5b in allergic airways. ( c – e ) Muc5ac messenger RNA increased 383-fold in OVA-challenged WT mice (+/+), but it was undetectable in Muc5ac knockout (−/−) mice ( c ), resulting in a 67% reduction in mucous metaplasia detected by periodic acid fluorescent Schiff’s staining ( d and e ). Scale bars, 20 μm ( a , b , d ). Mean, s.e.m. ( c and e ). * P <0.05 (one-tailed) by a unpaired t -test ( c and e ), with Welch’s correction for unequal variances in c . ND, not detected. Numbers in parentheses, ‘ N ’ mice. ‘Vol.’, volume. Dashed line in e , baseline in saline-challenged WT mice. Full size image Muc5ac is required for AHR to MCh in allergic mouse lungs To determine the consequences of disrupting Muc5ac expression on airflow obstruction, we assessed lung mechanical function and AHR to MCh. OVA challenge did not alter baseline lung resistance ( Supplementary Fig. 1a ), demonstrating that inflammatory and mucous metaplastic changes did not disrupt steady-state airflow measurably in this model of late-phase asthma. However, when exposed to MCh, OVA-challenged WT and heterozygous mice both demonstrated significant AHR. By contrast, Muc5ac −/− mice were protected ( Fig. 2a ; Supplementary Fig. 1b ). To confirm these findings, we also assessed AHR in C57BL/6 and BALB/c WT and congenic Muc5ac −/− mice exposed to aerosolized Aspergillus oryzae extract (AOE). AOE is a fungal allergen pertinent to human asthma that upon mucosal sensitization elicits strong asthma-like responses in mice [38] . In WT animals, AOE challenge caused AHR to MCh, but in both Muc5ac −/− lines, AHR was abolished ( Fig. 2b,c ; Supplementary Fig. 1b ). Importantly, protection occurred irrespective of C57BL/6 and BALB/c strain-specific airway- and tissue-localized pathophysiologies. To partition AHR on airway and tissue scales, we assessed lung mechanics by measuring input impedance. As reported previously [39] , AHR was strongly influenced by tissue resistance and elastance in C57BL/6 mice ( Fig. 3a ; Supplementary Fig. 2 ) and by tissue and central airway resistance in BALB/c mice ( Fig. 3b ; Supplementary Fig. 2 ); Muc5ac deficiency was protective irrespective of the background strain. Thus, in diverse models of allergic asthma, Muc5ac was required for AHR to MCh. 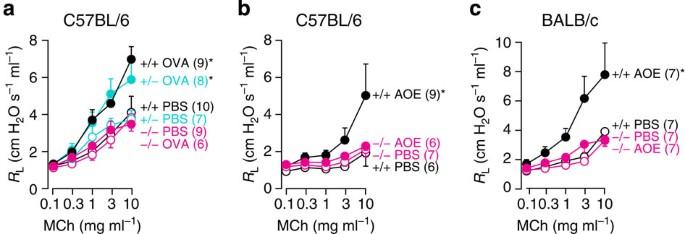Figure 2: Muc5ac is required for AHR to MCh. Lung resistance (RL) responses to MCh in WT (+/+, black),Muc5ac+/−(turquoise) andMuc5ac−/−(magenta) mice after saline (open circles), OVA (closed circles ina) orAspergillus oryzaeextract (AOE; closed circles inbandc). Mean, s.e.m. (a–c). *P<0.05 between slopes of best-fit regression lines by one-way ANOVA. Numbers in parentheses, ‘N’ mice. Figure 2: Muc5ac is required for AHR to MCh. Lung resistance ( R L ) responses to MCh in WT (+/+, black), Muc5ac +/− (turquoise) and Muc5ac −/− (magenta) mice after saline (open circles), OVA (closed circles in a ) or Aspergillus oryzae extract (AOE; closed circles in b and c ). Mean, s.e.m. ( a – c ). * P <0.05 between slopes of best-fit regression lines by one-way ANOVA. Numbers in parentheses, ‘ N ’ mice. 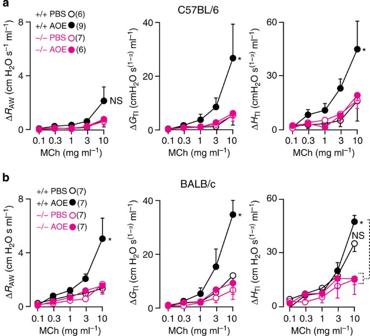Figure 3: Muc5ac mediates mouse strain-specific allergic airway pathophysiology. Conducting airway resistance (ΔRAW), tissue resistance (ΔGTI) and tissue elastance (ΔHTI) were measured using oscillatory mechanics to assess input impedance. (a) In WT C57BL/6 mice,Aspergillus oryzaeextract (AOE)-induced AHR (closed black circles) was dominated by changes in peripheral tissue mechanics (ΔGTIand ΔHTI) compared with changes inRAW. (b) In WT BALB/c mice, AOE-induced AHR (closed black circles) had central airway (ΔRAW) and tissue dominance (ΔGTI), whereas ΔHTIwas not significantly different following AOE (NS) in WT mice. In both congenic strains, responses were significantly blunted inMuc5ac−/−mice (closed magenta circles). Mean, s.e.m. *P<0.05 between slopes of best-fit regression lines by one-way ANOVA. ‘NS’, not significant. Numbers in parentheses, ‘N’ mice. Full size image Figure 3: Muc5ac mediates mouse strain-specific allergic airway pathophysiology. Conducting airway resistance (Δ R AW ), tissue resistance (Δ G TI ) and tissue elastance (Δ H TI ) were measured using oscillatory mechanics to assess input impedance. ( a ) In WT C57BL/6 mice, Aspergillus oryzae extract (AOE)-induced AHR (closed black circles) was dominated by changes in peripheral tissue mechanics (Δ G TI and Δ H TI ) compared with changes in R AW . ( b ) In WT BALB/c mice, AOE-induced AHR (closed black circles) had central airway (Δ R AW ) and tissue dominance (Δ G TI ), whereas Δ H TI was not significantly different following AOE (NS) in WT mice. In both congenic strains, responses were significantly blunted in Muc5ac −/− mice (closed magenta circles). Mean, s.e.m. * P <0.05 between slopes of best-fit regression lines by one-way ANOVA. ‘NS’, not significant. Numbers in parentheses, ‘ N ’ mice. Full size image Mucin secretion alone is not sufficient to cause AHR Because acute mucin secretion was required for AHR to MCh with no residual effect attributable to ASM hypercontractility ( Figs 2 and 3 ), we next determined whether mucin secretion was sufficient to acutely induce AHR independently of bronchoconstriction. In airway epithelial cells, P2Y 2 purinergic receptor stimulation is a major pathway for mucin secretion [40] . P2Y 2 receptors are activated by the endogenous agonists ATP and uridine triphosphate trisodium salt (UTP) [40] , [41] . ATP is rapidly dephosphorylated to adenosine, a signalling molecule that itself induces bronchoconstriction; ATP was thus inappropriate for these studies. Since UTP and its metabolites do not cause acute ASM contraction [42] , we challenged WT C57BL/6 mice with OVA or saline, and 72 h later we mechanically ventilated them and measured immediate changes in secretion and lung resistance in response to UTP. In OVA-challenged WT mice, although UTP rapidly stimulated secretion ( Fig. 4a,b ), there was no disruption of airflow ( Fig. 4c ). Thus, although Muc5ac was critical for allergic AHR in the presence of ASM-mediated bronchoconstriction following MCh, UTP-induced mucin secretion alone did not evoke an AHR response. 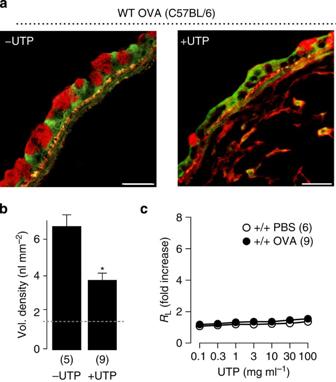Figure 4: Acute mucin secretion does not cause AHR. WT mice were OVA or PBS challenged, and then anaesthetized, ventilated and exposed to UTP (0.1–100 mg ml−1) or vehicle (saline). (a) In OVA-challenged lungs fixed immediately after dose–response tests, there was an acute decrease in periodic acid fluorescent Schiff’s (PAFS) staining in UTP (right panel) compared with vehicle-(‘−UTP’, left panel) treated mice, demonstrating acute UTP-induced secretion. Scale bars, 20 μm. (b) Quantitation of UTP-induced changes in PAFS staining in OVA-challenged mice. (c) No effect of UTP onRLin either PBS- or OVA-challenged WT mice. Mean, s.e.m. inbandc. Numbers in parentheses, ‘N’ mice. ‘Vol.’, volume. Dashed line inb, baseline in saline-challenged WT mice. *P<0.05 by thet-test. Figure 4: Acute mucin secretion does not cause AHR. WT mice were OVA or PBS challenged, and then anaesthetized, ventilated and exposed to UTP (0.1–100 mg ml −1 ) or vehicle (saline). ( a ) In OVA-challenged lungs fixed immediately after dose–response tests, there was an acute decrease in periodic acid fluorescent Schiff’s (PAFS) staining in UTP (right panel) compared with vehicle-(‘−UTP’, left panel) treated mice, demonstrating acute UTP-induced secretion. Scale bars, 20 μm. ( b ) Quantitation of UTP-induced changes in PAFS staining in OVA-challenged mice. ( c ) No effect of UTP on R L in either PBS- or OVA-challenged WT mice. Mean, s.e.m. in b and c . Numbers in parentheses, ‘ N ’ mice. ‘Vol.’, volume. Dashed line in b , baseline in saline-challenged WT mice. * P <0.05 by the t -test. Full size image Allergic inflammation fails to drive AHR in Muc5ac null mice Type-2 inflammation is critical for AHR in allergic mouse models [30] , [31] . Given the essential role for Muc5ac in AHR identified here ( Figs 2 and 3 ), and the requirement for Muc5b in inflammatory cell clearance [25] , we determined whether Muc5ac expression mediated AHR by modulating allergic inflammation. Compared with saline-challenged mice, there were significant increases in leukocyte numbers that varied with environmental exposure (OVA versus AOE) and genetic diversity (C57BL/6 versus BALB/c) ( Supplementary Table 1 ). In WT C57BL/6 mice, there was an 8.5-fold difference in eosinophilic responses to OVA and AOE; between WT BALB/c and C57BL/6 strains, there was a 9.7-fold difference in eosinophil numbers in response to AOE ( Fig. 5 ). However, between WT and Muc5ac −/− mice in each of these groups, eosinophilic inflammation was not significantly different ( Fig. 5 ; Supplementary Fig. 3 ; Supplementary Table 1 ). Thus, full protection from AHR in the absence of Muc5ac occurred although asthma-like allergic inflammation was sustained. 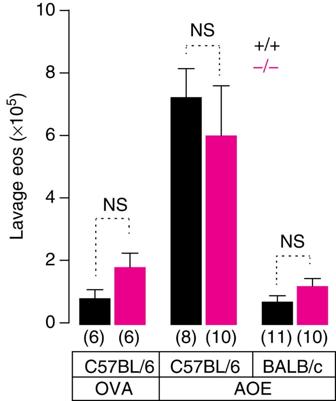Figure 5: Muc5ac deficiency does not reduce allergic inflammation. WT (black) andMuc5ac−/−(magenta) mice had similar numbers of eosinophils in lung lavage fluid irrespective of OVA orAspergillus oryzaeextract (AOE) antigen challenge or strain background variables. For all groups, saline-challenged mice had <104eosinophils in lung lavage fluid (seeSupplementary Table 1). Mean, s.e.m.N=6–11 mice per group. Figure 5: Muc5ac deficiency does not reduce allergic inflammation. WT (black) and Muc5ac −/− (magenta) mice had similar numbers of eosinophils in lung lavage fluid irrespective of OVA or Aspergillus oryzae extract (AOE) antigen challenge or strain background variables. For all groups, saline-challenged mice had <10 4 eosinophils in lung lavage fluid (see Supplementary Table 1 ). Mean, s.e.m. N =6–11 mice per group. Full size image Reduced heterogeneous airway closure in Muc5ac null mice Since AHR was abolished in Muc5ac −/− mice although inflammation remained intact, we hypothesized that AHR was mediated by physical obstruction of the airway lumen by Muc5ac. Obstruction could result from uniformly thickened mucus causing an increase in resistance to airflow via homogeneous changes in mean airway lumen diameter. Alternatively, obstruction could result from non-uniform mucous aggregates causing an increase in resistance to airflow via heterogeneous occlusion and airway closure ( Fig. 6a ). To compare these, AOE-challenged WT and Muc5ac −/− mice were mechanically ventilated and treated with increasing doses of MCh as shown in Fig. 2 . During peak changes in resistance following 10 mg ml −1 MCh, lungs were fixed transmurally with methacarn to preserve airway geometry and enable quantification of secreted mucus in situ [43] . 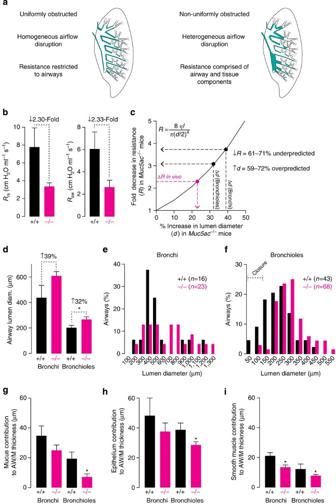Figure 6: Muc5ac deficiency protects against heterogeneous airflow obstruction. (a) Models of the effects of uniform versus non-uniform obstruction on airflow. (bandc) Changes in peak total lung and airway resistances (ΔR) following 10 mg ml−1MCh in WT andMuc5ac−/−mice (n=7 per genotype) (b) were fit to Poiseuille’s law (equation inc) to predict changes in airway lumen diameter (magenta point and dashed arrow). Viscosity (η) and length (l) were held constant. (d–f) Mean (d) and distributions (e,f) of airway lumen diameters measured in methacarn-fixed lungs; changes in mean lumen diameter were also fit to the equation inc(black points and dashed arrow). (g–i) Contributions of mucus, airway epithelium and smooth muscle to changes in composite airway wall/mucus (AW/M) thickness. Mean, s.e.m. inb,dandg–i.xaxis labels bin maximum values ineandf.N=4 WT and 5Muc5ac−/−mice. *P<0.05 by at-test. Figure 6: Muc5ac deficiency protects against heterogeneous airflow obstruction. ( a ) Models of the effects of uniform versus non-uniform obstruction on airflow. ( b and c ) Changes in peak total lung and airway resistances (Δ R ) following 10 mg ml −1 MCh in WT and Muc5ac −/− mice ( n =7 per genotype) ( b ) were fit to Poiseuille’s law (equation in c ) to predict changes in airway lumen diameter (magenta point and dashed arrow). Viscosity ( η ) and length ( l ) were held constant. ( d – f ) Mean ( d ) and distributions ( e , f ) of airway lumen diameters measured in methacarn-fixed lungs; changes in mean lumen diameter were also fit to the equation in c (black points and dashed arrow). ( g – i ) Contributions of mucus, airway epithelium and smooth muscle to changes in composite airway wall/mucus (AW/M) thickness. Mean, s.e.m. in b , d and g – i . x axis labels bin maximum values in e and f . N =4 WT and 5 Muc5ac −/− mice. * P <0.05 by a t -test. Full size image We generated a model of homogenous obstruction by fitting changes in resistance and airway lumen diameter to Poiseuille’s law. In AOE-challenged Muc5ac −/− mice, resistance ( R ) to airflow decreased 2.3-fold ( Fig. 6b ). Assuming laminar flow, Poiseuille’s law predicts a 23% increase in mean lumen diameter uniformly ( Fig. 6c , magenta dashed line). However, our histological measurements showed that mean lumen diameters improved by 39% and 32% in bronchi and bronchioles, respectively ( Fig. 6d ). If applied to the model above, airflow resistances would be three- to fourfold improved ( Fig. 6c , black lines), but they were not. Thus, a model in which the prevention of AHR in Muc5ac −/− mice was the result of protection from uniform mucus thickening and homogenous airflow obstruction is incongruent with our observations. Indeed, the poor fit of the findings above, the anatomically diverse responses observed in our AHR studies ( Fig. 3a,b ) and previous data from murine and computational models [2] , [8] more strongly support heterogeneous obstruction as the major determinant of AHR. To determine whether Muc5ac-mediated heterogeneous obstruction contributes to AHR, we analysed the distributions of individual airway lumen sizes relative to their anatomical locations. We observed non-uniform distributions of lumen sizes. In Muc5ac −/− lungs, there was a rightward shift in the distribution of airway lumen sizes compared with WT ( Fig. 6e,f ), which was consistent with protection from AHR. Furthermore, in WT mice, we also observed markedly greater proportions of bronchiolar airways with diameters of ≤100 μm ( Fig. 6f ), a measurement consistent with a previously calculated threshold for airway closure [8] . Because components such as the epithelial and ASM layers and secreted mucus can all influence airway closure, we next determined how these were affected in Mu5ac −/− mice. In our functional studies, epithelial mucin production/secretion and ASM contraction were both required for AHR as shown in Figs 2 , 3 , 4 . We thus compared the specific contributions of secreted mucin, epithelial thickening and ASM to anatomically localized changes in airway sizes. In bronchi, overall airway diameter (including ASM, epithelium, mucus and lumen) was 539±78 μm in WT mice and 683±31 μm in Muc5ac −/− mice ( P =0.051, one-tailed t -test), and in the bronchioles, these values were 274±15 μm and 310±22 μm, respectively ( P =0.096, one-tailed t -test). Although not statistically significant as a combined group, these data suggested that secreted Muc5ac in the airway lumen could have some effect(s) on the behaviour of underlying tissues. We therefore derived a measure of composite airway wall/mucus thickness by subtracting airway lumen diameters ( Fig. 6d ) from overall airway diameters. In the bronchi, this was not significantly different between WT and Muc5ac −/− mice (103±21 versus 76±9 μm, respectively; P =0.124, one-tailed t -test). By contrast, in the bronchioles, differences in composite airway wall/mucus thickness were significant (71±14 μm in WT versus 44±10 μm in Muc5ac −/− ; P =0.006, one-tailed t -test). Mucus contribution to composite airway wall/mucus thickness was reduced in Muc5ac −/− mice compared with WT as expected, since a major mucin component was missing ( Fig. 6g ). However, there were also significant differences in epithelial tissue and ASM components ( Fig. 6h,i ). Epithelial hypertrophy is directly related to mucin production [9] , so its contribution was also predictable ( Fig. 6h ). By contrast, the effect of Muc5ac deficiency on the contribution of ASM, which was significantly lower in Muc5ac −/− bronchi and bronchioles, was surprising ( Fig. 6i ). Collectively, these findings reinforce the concept AHR is caused by contractile and non-contractile factors that contribute interdependently. Since AHR in allergic mouse lungs was dependent on a combination of ASM contraction and Muc5ac secretion ( Figs 2 , 3 , 4 ), and since changes in airway structure and function did not fit models of homogenous changes in airflow, these findings further support the hypothesis that epithelial Muc5ac secretion during MCh-induced ASM constriction causes the formation of mucous plugs that potentiate heterogeneous airflow disruption. Muc5ac mediates heterogeneous mucous occlusion in mice In WT airways, mucous plugs were present and Muc5ac was abundant ( Fig. 7a ); in Muc5ac −/− airways, plugs were infrequent and mucus was sparse ( Fig. 7b ). Throughout the lungs, mean lumen mucin volume density, a homogeneous measure of mucous content across airway surfaces, was reduced by 32% ( Table 1 ). Thus, as with lumen diameter, assuming uniform mucus accumulation across all airway surfaces and fitting these to Poiseuille’s law results in changes in resistance that exceed those observed experimentally. 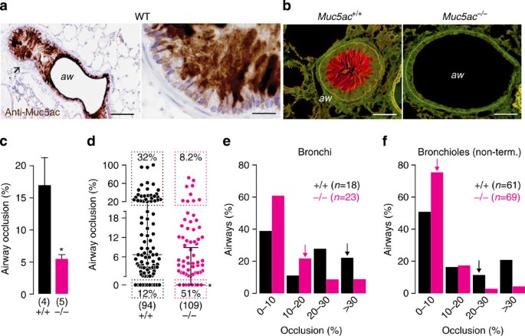Figure 7:Muc5ac deficiency reducesmucousplugging. (aandb) Inhaled MCh caused mucous plugging in WT allergic mouse airways (aw). Muc5ac protein (a) and PAFS staining (b) in AOE-challenged WT (Muc5ac+/+) andMuc5ac−/−mouse airways. Arrow ina, region is shown at a higher magnification in the right panel. (c–f) Extent and distribution of mucous plugging. Mean occlusion per mouse across all measured airways (c). Distribution of the extent (d) and localization (eandf) of occlusions. Arrows ineandf, starts of upper quartiles. Scale bars, 100 and 20 μm (a); 50 μm (b). Mean, s.e.m. (c). Median quartiles (d). *P<0.05 (one-tailed) by an unpairedt-test (c) and the Mann–Whitney test (d). Numbers in parentheses, ‘N’ mice (c), ‘N’ airways (d–f). Figure 7: Muc5ac deficiency reduces mucous plugging. ( a and b ) Inhaled MCh caused mucous plugging in WT allergic mouse airways (aw). Muc5ac protein ( a ) and PAFS staining ( b ) in AOE-challenged WT ( Muc5ac +/+ ) and Muc5ac −/− mouse airways. Arrow in a , region is shown at a higher magnification in the right panel. ( c – f ) Extent and distribution of mucous plugging. Mean occlusion per mouse across all measured airways ( c ). Distribution of the extent ( d ) and localization ( e and f ) of occlusions. Arrows in e and f , starts of upper quartiles. Scale bars, 100 and 20 μm ( a ); 50 μm ( b ). Mean, s.e.m. ( c ). Median quartiles ( d ). * P <0.05 (one-tailed) by an unpaired t -test ( c ) and the Mann–Whitney test ( d ). Numbers in parentheses, ‘ N ’ mice ( c ), ‘ N ’ airways ( d – f ). Full size image Table 1 Measurements of secreted mucus in mice during bronchoconstriction. Full size table We thus determined the extent and distribution of mucous occlusion percentage, a sensitive measure of the fractional volume of airspaces occupied by mucus. This was used previously to quantify the prevalent but heterogeneous airway plugging observed in fatal asthma, which showed that >98% of airways in these patients were occluded with mucus by 20% or more [15] . In Muc5ac −/− airways, overall mean lumen occlusion percentage was reduced by ~60% ( Table 1 ; Fig. 7c ). Similar to human asthma [15] , plugging was also heterogeneous in mice ( Fig. 7d ). In WT airways, median occlusion was 6.7% compared with 0% in Muc5ac −/− airways. Furthermore, in WT mice only 12% of airways were occlusion free, and 32% were occluded by ≥20%. In Muc5ac −/− mice, 51% of airways were occlusion free, and only 8.2% were occluded by ≥20%. To further dissect the sources of heterogeneous obstruction, we determined the distribution of occlusions by airway generation. In WT mice, occlusions of ≥20% were common in axial bronchi (50% of airways) and bronchioles (31% of non-terminal airways) ( Fig. 7e,f ). In Muc5ac −/− mice, occlusions of ≥20% were present in only 17.4% of axial bronchi (2.7-fold reduction) and 7.2% of bronchioles (4.6-fold reduction). Thus, disruption of the Muc5ac gene in mice resulted in protection from a heterogeneous airway plugging phenotype that was similar to the pathology observed in fatal human asthma [15] . AHR in asthma is currently thought to result primarily from inflammation-triggered ASM hypercontractility [1] . However, there is growing evidence that in addition to ASM-driven narrowing, obstruction is also mediated by significant non-contractile factors [2] , [4] , [8] , [44] . Here we report that in allergically inflamed mouse lungs, Muc5ac is an essential non-contractile mediator of AHR. These findings have important implications with respect to mechanisms of asthma pathophysiology. They could also inform the development of more effective treatments that target MUC5AC. These could especially benefit patients in whom bronchodilators or corticosteroids are ineffective [1] , [45] . In our studies, mucin secretion and ASM contraction were both required for AHR. Although there were C57BL/6 and BALB/c strain-specific differences between central airway and peripheral tissue responses, there was no residual AHR to MCh in Muc5ac −/− mice at whole-lung or partitioned airway and tissue scales. Thus, our data challenge the notion that AHR in allergic asthma is dominated by exaggerated ASM contraction. That dogma is grounded on studies showing ASM hypertrophy in pathological tissues, hypercontractility of excised ASM from asthma patients and on protection provided by bronchodilating β-agonist treatments [1] . Such findings show association and suggest necessity for ASM hypercontractility in AHR, but they do not prove its sufficiency. Our studies also showed that inducing mucin secretion without bronchoconstriction did not evoke AHR. Thus, in mice, while ASM contraction and mucin secretion are both necessary for acute AHR, neither alone is sufficient. Rather, ASM contraction and mucin secretion mediate AHR cooperatively. These findings highlight the need to better understand coordinated contractile and non-contractile mechanisms of airflow obstruction in asthma [2] . In addition to finding that ASM contraction and Muc5ac secretion were both required for AHR, we also found an apparent interdependence between mucus secretion and ASM-mediated airway constriction. Airway diameters and ASM thickness were both significantly reduced in allergic Muc5ac −/− lungs after MCh ( Fig. 6 ). This may reflect effects of mucus secretion on airway surface tension and the propensity for airway closure, or it may demonstrate the ability of airways with less mucus to remain open following deep lung inflation manoeuvres that are administered between MCh doses in our experimental set-up. In asthma patients, these could affect the ability of deep breaths to maintain open airways. Alternatively, during dose–response tests in our studies, enhanced passage of aerosolized MCh through open airways in Muc5ac −/− mice could have increased its deposition in the terminal bronchioles, which have little to no smooth muscle or mucin expression and thus contribute minimally to AHR. Lastly, changes in ASM constriction could have been related to changes in ASM hypertrophy in allergic Muc5ac −/− mice. However, this is unlikely since the total amount of ASM was not different between allergic WT and Muc5ac −/− mice ( Supplementary Table 2 ). Nonetheless, further investigation is needed to determine the potential significance and mechanisms of these intriguing interactions between ASM and non-contractile components. To this end, other non-contractile factors of AHR have been studied [2] , [3] , [8] . Plasma extravasation and fibrin accumulation can reduce airway liquid surface tension and cause acute airway closure [3] . Studies in animal and computational models present this alternative to ASM dominance as heterogeneous closure occurring via ‘sudden liquid bridge formation’ [2] , [8] . Our findings are consistent with this conceptual framework, which we advance by defining Muc5ac as a key molecular mediator. Indeed, it is plausible that aqueous-soluble factors become enriched within hydrated and heterogeneously distributed Muc5ac-containing mucous aggregates. Alternatively, each could occur independently yet synergize to mediate airway closure during bronchoconstriction. Our studies also demonstrated that Muc5ac mediates AHR independently of the degrees of allergic inflammation. Differences in genetic and stimulus-dependent allergic inflammation were striking ( Fig. 5 ; Supplementary Fig. 3 ; Supplementary Table 1 ). However, although inflammation is critical for allergic AHR [30] , [31] , and secreted mucins can modulate immune function and resolve inflammation [25] , [26] , [46] , eosinophils in OVA- and AOE-challenged Muc5ac −/− lungs did not differ from WT ( Fig. 5 ). By contrast, mucous plugs throughout Muc5ac −/− airways were significantly reduced in abundance and severity ( Fig. 7 ). Thus, protection from AHR was mediated not by altered inflammation but through reduced plug formation: in constricting airways, acute physical obstruction caused by Muc5ac was essential for AHR. This segregation between Muc5ac function and preserved type-2 inflammation is consistent with in vivo findings in nematode-infected mice. ‘Allergic’ type-2 inflammation stems from off-target anti-helminth responses. In nematode-infected Muc5ac −/− mice, although intestinal type-2 inflammation is sustained, animals do not effectively control infections in the absence of Muc5ac [37] . Rather than affecting inflammation, the type-2 inflammation effector Muc5ac (but not the homeostatic intestinal mucin Muc2) directly impairs worm viability [37] . It remains to be determined whether the mechanisms by which Muc5ac selectively inhibits worm growth also promote mucus aggregation and plugging in the airways. Indeed, biochemical/biophysical mechanisms by which secreted mucus occludes airways in asthma are poorly understood. Our current understanding of mucins in asthma is largely limited to anecdotal evidence of altered physical properties [19] , to associations drawn from pathological studies showing increased goblet cell numbers and mucin contents in biopsies from a wide range of disease severities [4] , [47] and to pervasive airway plugging in autopsy specimens obtained from fatal cases [15] , [16] , [17] . Some studies do show that patients have persistently abnormal mucus and mucociliary clearance [4] , [11] , [19] , [20] , [23] , [48] , [49] . However, the obstructive consequences of mucin secretion in AHR and non-fatal exacerbations have remained unclear. This may be due in part to a lack of appreciation of interrelated ASM contractile and epithelial secretory processes. MCh induces both ASM contraction and epithelial mucin secretion [21] , [22] . In the airways, mucins become hydrated [50] , swelling to produce a thick gel that amplifies the obstructive effects of narrowing initiated by ASM [2] , [4] . Applying strategies that combine relaxing ASM with reducing mucin production and secretion and/or enhancing mucociliary clearance could improve disease treatment. While potentially beneficial, clearance-enhancing mucolytics and expectorants have been disregarded as asthma treatments. At achievable doses, existing therapies such as hypertonic saline and N -acetylcysteine show poor efficacy and tolerability, because the high concentrations that are needed to clear mucous plugs are irritating and cause bronchoconstriction [4] , [51] , [52] , [53] . For example, although N -acetylcysteine is the only Food and Drug Administration-approved reducing agent available as an inhaled adjunct mucolytic, clinical data do not support its use [54] , reflecting its low mucolytic activity at high mucin concentrations [55] , [56] and at a neutral airway pH (7.14 in mice [57] ). We speculate that improved inhaled mucolytic agents can reduce plugging and AHR in asthma. However, it will be critical for any strategy that reverses or prevents obstruction, to do so safely while also protecting mucous-mediated defence. Muc5ac is one of two polymeric mucins that are the predominant glycoproteins in airway mucus. The other, Muc5b, is expressed abundantly at baseline and remains present following allergic inflammation in mice ( Fig. 1a,b ). Muc5b is critical for homeostatic defence. Muc5b −/− , but not Muc5ac −/− , mice have severely impaired mucociliary clearance functions, resulting in accumulated particles and bacteria in the airways, and ultimately in death due to uncontrolled infection [25] . In humans with asthma, as MUC5AC expression increases, MUC5B expression either remains stable or decreases markedly [10] , [12] , with divergent MUC5AC : MUC5B expression ratios associated with worse AHR [10] . Thus, targeting MUC5AC, while preserving or enhancing MUC5B, should be considered for any improved mucolytic therapies. Two possible means for controlling the effects of MUC5AC on AHR are through targeting gene expression mechanisms or the glycoprotein itself. Critical expression signals include IL-13 and epidermal growth factor receptor ligands [34] , [35] , [36] . A monoclonal anti-IL-13 antibody has shown promise in early human trials [29] , and a small-molecule inhibitor of MAPK13 was effective in allergic mice [58] . However, a recent trial of epidermal growth factor receptor blockade in chronic obstructive pulmonary disease (COPD) failed, because at doses that achieved minimal changes in mucin production, adverse effects occurred [59] . Transcriptional control of MUC5AC/Muc5ac gene expression through regulators including SPDEF (SAM pointed domain-containing Ets transcription factor), Notch and hypoxia-inducible factor-1 (refs 24 , 60 , 61 , 62 ) have also been identified, but they are not currently targetable. As an alternative to controlling gene expression, more selective results could potentially be yielded by disrupting the secreted MUC5AC polymer or by blocking its assembly. Recent studies have revealed mechanisms for controlling mucin disulfide bond-mediated polymerization [63] and patterns of selective mucin glycosylation [23] , [49] . These may provide better targets for preventing mucus aggregation and airway plugging acutely. Specifically, by determining which glycan or oligomerization mechanisms are specific for MUC5AC versus MUC5B, novel strategies could be designed to reduce AHR by selectively inhibiting MUC5AC-mediated plugging while maintaining MUC5B-mediated airway defence. Future studies are directed at investigating these possible mechanisms. Since excessive MUC5AC is also a common problem in airway diseases such as COPD and cystic fibrosis, whose inflammation and MUC5AC gene induction pathways differ significantly from allergic asthma, targeting the physical glycoprotein and polymeric properties of MUC5AC could have broader therapeutic applications. Experimental animals Studies were performed with approval of the animal care and use committees of the University of Colorado (approval number 97412(01)E) and the MD Anderson Cancer Center (approval numbers 05-04-046, 05-05-04334 and 00001214-RN00). Muc5ac −/− mice were generated previously [37] . Mice were backcrossed onto congenic C57BL/6 and BALB/c lines using marker-assisted analysis at the MD Anderson Research Animal Support Facility-Smithville, Animal Genetics Services lab. After achieving 100% carriage of 77 C57BL/6 and 82 BALB/c strain-specific markers, lines were backcrossed 3–5 additional generations. Mice were either bred as homozygous nulls or heterozygotes. C57BL/6 and BALB/c mice from the Jackson Labs (Bar Harbor, ME) were used for congenic backcrossing and as WT controls. Male and female mice were used starting at 7–8 weeks age. Before and after exposures, mice were housed under specific pathogen-free conditions in ventilated cages (≤5 mice per cage) with a 12-h light/dark cycle and with food and water available ad libitum . Mice were placed into experimental and control groups chronologically. Ovalbumin- and A. oryzae induced lung inflammation For studies in OVA-challenged mice, animals were sensitized intraperitoneally (i.p.) with 4 weekly injections of 20 μg OVA, 2.25 mg alum in saline (Sigma, St Louis, MO). Seven days after the last injections, sensitized mice were then exposed to 5 ml of a 2.5% (w/v) OVA aerosol delivered until the full volume was administered [9] . For AOE challenge, mice were exposed by the nose-only inhalational challenge. AOE is a commercially available fungal protease/peptidase complex produced by submerged fermentation of A. oryzae (catalogue no. P6110 Sigma). Although marketed as a ‘protease,’ our own microscopic analysis shows that it is a crude extract rich in fungal particles, although no live organisms were detected when samples were cultured. In addition, endotoxin levels were <50 units ml −1 (Endosafe-PTS, Charles River Laboratories, Wilmington, MA). AOE was used previously to elicit allergic inflammation in mice following bolus intranasal application [38] . For aerosol exposures here, a 5-ml volume of a 10% v/v solution of AOE was made in PBS containing 2.5% w/v OVA (Sigma) and 1% v/v antifoam A (Sigma). Aerosols were generated using an Ultravent jet nebulizer, which when driven at 30 psi, generates particles with a mean mass aerodynamic diameter of <1 μm [64] . In mice, >80% of the particles generated are respirable and deposit in the lower airways efficiently [64] . Exposures were made in custom-built nose-only chambers and lasted until a 5-ml volume was delivered (40–45 min). Mice were AOE challenged once weekly for 4 weeks. Allergic inflammation was confirmed by lung lavage and Giemsa staining. Muc5ac messenger RNA levels were determined by quantitative PCR as described previously [24] . Airway hyperreactivity Lung function was measured 72 h post OVA challenge or 48 h post AOE challenge using a flexiVent (Scireq, Montreal, Quebec, Canada). Mice were anaesthetized with 2.0 g kg −1 urethane (i.p.). This was sufficient to provide up to 4 h of sedation, although experiments lasted only 20–40 min. Mice were tracheostomized with a blunt beveled 18 G Luer stub adapter. Once ventilated (150 breaths per min, 10 ml kg −1 , against 3 cm H 2 O positive end expiratory pressure), mice were paralysed by continuous infusion of succinylcholine chloride (10 μg g −1 min −1 , i.p.). Baseline total lung resistance ( R L ) using a single-compartment model and the input impedance parameters, Newtonian (airway) resistance ( R AW ), tissue resistance ( G TI ) and tissue elastance ( H TI ) were determined. Changes in R L , R AW , G TI and H TI in response to successive, increasing doses of MCh chloride (Sigma, Cat no. A2251; 0.1–10 mg ml −1 ) or UTP (Sigma, Cat no. 94370; 0.1–100 mg ml −1 ) administered by an in-line ultrasonic nebulizer were assessed. Heart rates were monitored by electrocardiogram. At 10 mg ml −1 MCh, heart rates often fell below 200 beats per min and did not recover. At this point, no further dose–response measurements were made. Mucin production and secretion To assess mucin production, mouse lungs were fixed by intratracheal formalin administration and stained using periodic acid fluorescent Schiff’s (PAFS) to assess and quantify intracellular glycoconjugates [9] , [65] . To assess secretion, WT C57BL/6 mice were OVA challenged, ventilated on a flexiVent and exposed to inhaled UTP to induce secretion (0.1–100 mg ml −1 ) or inhaled saline to control for ventilator- or vehicle-induced secretion (seven doses repeated over the same intervals used for UTP). After UTP or saline exposures, lungs were immediately fixed intratracheally with formalin. Acute mucin secretion in airway tissues was assessed by measuring changes retained in PAFS-positive contents. Secretion was defined as decreased staining due to acute depletion of intracellular stores in UTP versus saline-treated animals. Mucous plugging and airway measurements Tissues were fixed by adapting a method previously used to preserve colonic mucus using methanol-based Carnoy’s fixative (methacarn) [43] . Methacarn is a highly permeant non-crosslinking preservative that rapidly penetrates tissues transmurally while minimizing mucus disruption and tissue shrinkage [43] . Animals were carried through full dose–response curves. During peak increases in R L following 10 mg ml −1 MCh, mice were rapidly euthanized by anaesthetic overdose and cessation of mechanical ventilation. Mice remained connected to the ventilator, which by default stopped at end expiration (3 cm H 2 O positive end expiratory pressure). Skin covering the lower sternum was removed, and 400 μl of methacarn was injected into the pleural space. The trachea was ligated immediately below the tracheal cannula. These steps took less than 15 s, thus minimizing changes in airway constriction and mucus transport. Lungs were fixed in situ for 30–60 min, then removed and immersion fixed with the trachea still ligated for 24–48 h in methacarn at 4 °C. Tissues were transferred to 100% methanol (changed twice over a 48-h period). While remaining fully immersed in methanol, left lungs were sectioned into uniform 1.92-mm-thick filets and imaged to calculate volume by Cavalieri estimation (319±31 and 322±24 mm 3 for WT and Muc5ac −/− mice, respectively). Tissues were then paraffin processed and sectioned (5 μm thickness). Histological assessments were made using alcian blue-periodic acid Schiff's (AB-PAS) and periodic acid fluorescent Schiff's (PAFS) to assess total mucin, Muc5ac (clone 45M1, 1:100 dilution), and MUC5B (custom polyclonal antisera, 1:2,000) production [37] , [65] , [66] . Intracellular mucin content levels and the extent of mucous plugging were examined by systematic uniform random sampling [67] . Stained slides were scanned by two blinded investigators using an Olympus BX63 microscope and cellSens software (Olympus USA, Center Valley, PA). At least five axial bronchi per mouse were analysed. For non-axial ‘bronchiolar’ airways, samples were analysed by selection of every fifth × 20 image in a continuous x -/ y - map of all lung samples per slide. Mucin and airway area were calculated using point-grid counting. Basement membrane length and airway circumferences were measured in cellSens. Data were calculated as volume densities (volume per unit surface area of basement membrane) [9] , [65] and as extracellular mucous volume fractions relative to lung and airway volumes (multiplied by 100 to express as % occlusion) [67] . Statistical analyses All statistical analyses were performed using GraphPad Prism 5.04 with a P value cutoff of 0.05 considered significant. Inflammation, mucin production and mucin secretion data were compared between groups using unpaired one-way Student’s t -tests, with corrections made for unequal variances (Welch’s), or non-Gaussian distribution (Mann–Whitney) where appropriate. For multiple comparisons, analysis of variance (ANOVA) with a Dunnett post hoc correction or Kruskal–Wallis test for non-Gaussian distribution was used. For dose–response tests, curves were compared using ANOVA for repeated measures, and using ANOVA with a Dunnett post hoc correction to compare slopes after linear regression against log-transformed MCh doses. Both analyses of dose–response tests provided congruent results. Sample sizes were chosen based on the numbers of WT saline versus allergic mice required to achieve a statistically significant difference. How to cite this article: Evans, C. M. et al . The polymeric mucin Muc5ac is required for allergic airway hyperreactivity. Nat. Commun. 6:6281 doi: 10.1038/ncomms7281 (2015).